A visible dominant marker for insect transgenesis Transgenesis of most insects currently relies on fluorescence markers. Here we establish a transformation marker system causing phenotypes visible to the naked eye due to changes in the color of melanin pigments, which are widespread in animals. Ubiquitous overexpression of arylalkylamine- N -acetyl transferase in the silkworm, Bombyx mori , changes the color of newly hatched first-instar larvae from black to a distinctive light brown color, and can be used as a molecular marker by directly connecting to baculovirus immediate early 1 gene promoter. Suppression of black pigmentation by Bm- arylalkylamine- N -acetyl transferase can be observed throughout the larval stages and in adult animals. Alternatively, overexpression in another gene, B. mori β-alanyl-dopamine synthetase ( Bm-ebony ), changes the larval body color of older instars, although first-instar larvae had normal dark coloration. We further show that ectopic Bm- arylalkylamine- N -acetyl transferase expression lightens coloration in ladybird beetle Harmonia axyridis and fruit fly Drosophila melanogaster , highlighting the potential usefulness of this marker for transgenesis in diverse insect taxa. Genetic modification of insects is an essential and basic technique for studying developmental biology, as well as for applications such as pest control and recombinant protein production [1] . Transgenic techniques have been developed for many dipterans and lepidopteran insects [2] , [3] , and also for insects in other orders such as the red flour beetle Tribolium castaneum [4] , the ladybird beetle Harmonia axyridis [5] , the sawfly Athalia rosae [6] and the cricket Gryllus bimaculatus [7] . In Drosophila melanogaster , transgenic flies are generally identified by mutant-based genetic markers with visible phenotypes (for example, the white gene for eye pigmentation) [8] . However, most insect species do not have a set of suitable recipient mutant strains and the functional transgene to rescue the phenotype. Instead, fluorescence markers such as 3xP3-enhanced green fluorescent protein (EGFP), which drives the eye-specific expression of green fluorescent protein, are used [9] , [10] , [11] , [12] . As this transgene is dominant, it is especially useful for nontraditional model insects. However, screening under a fluorescence microscope is a laborious procedure for large-scale projects, and insect eyes normally have dark pigmentation, which makes detecting fluorescence difficult. Thus, the development of a dominant visible marker applicable to various strains would be beneficial for studies of non-Drosophila insects. For transgenic screening, it would be convenient if the altered phenotype could be easily identified externally at an early developmental stage. Suitable characteristics include unique pigmentation of eggs or neonatal larvae. One of the major pigments in insects is melanin, which is usually black or brown in color and is widespread in the exoskeletal cuticle [13] , [14] , [15] , [16] , [17] , [18] , [19] . Melanin-related pigments are mainly derived from dopamine [18] , [20] , [21] , which is synthesized from tyrosine by the enzymes tyrosine hydroxylase and dopa decarboxylase. Besides black and brown melanin pigments, dopamine is involved in the synthesis of light-coloured pigments and also in sclerotization. N -β-alanyl-dopamine (NBAD), a derivative of dopamine, is a precursor for the yellow/red cuticular pigments of Drosophila [18] and the larva of swallowtail butterfly, Papilio xuthus [15] , and for NBAD- o -quinone, which crosslinks cuticle proteins in sclerotization [22] , [23] . Another derivative of dopamine, N -acetyl-dopamine (NADA), is a precursor for NADA- o -quinone, which is also involved in sclerotization of transparent or very light-coloured cuticles [22] , [23] , [24] . Dopamine is converted to NBAD by the β-alanyl-dopamine synthetase encoded by ebony gene, whereas NADA is synthesized from dopamine by arylalkylamine- N -acetyl transferase (aaNAT) activity. The ebony mutant of Drosophila has darker overall coloration than wild type, and the ectopic expression of Dm-ebony changes the dark coloration of the adult abdomen to yellow [18] . In the silkworm Bombyx mori , the mutant allele of Bm-ebony is called sooty , which displays a distinct black pupal coloration instead of the normal light brown color [16] . The larvae and adults of sooty have a smoky color, which is less conspicuous than in pupae. The identity of the gene responsible for aaNAT activity in cuticle sclerotization is less clear. In insects, aaNAT activity is not only involved in sclerotization, but also in neurotransmitter catabolism and melatonin precursor formation [25] , [26] , [27] , [28] , [29] , [30] , [31] , [32] . Two aaNAT genes have been identified in Drosophila [25] , [26] , one of which is expressed in the brain. However, their involvement in sclerotization has not been reported, leaving open the possibility that an unidentified aaNAT enzyme may be involved in sclerotization in this insect. From the recent results of in vitro aaNAT activity analysis, aaNAT 1 and aaNAT 2 are assumed to be involved in sclerotization, and neurotransmitter inactivation in Aedes aegypti [33] . In B. mori , only one aaNAT gene, Bm-aaNAT has been characterized [28] . Notably, the mutant allele melanism ( mln ) does not display serious defects in sclerotization, but the adult shows darker overall pigmentation, and larvae show dark pigmentation in the head, forelegs and tail spot [34] , [35] . However, no reports exist for phenotypic effects of the mln mutant in the pupa and most parts of the larval epidermis [34] , [35] . Several aaNAT -like genes have been predicted in the B. mori genome based on sequence similarity [35] , which suggests that some of them may function in sclerotization in different regions and stages. As the substrates of aaNAT include dopamine [27] , [31] , it may be able to interfere with the synthesis of the dark dopamine-melanin. However, ectopic expression of aaNAT has never been tested in vivo in insects for converting dopamine to NADA. In silkworms, the neonatal larvae are black in color due to melanin, and are traditionally called ‘ants’ in Japanese. The development of a transgene that could change the color of the cuticle in insects of this stage in a dominant manner would be beneficial for the production and maintenance of transgenic silkworm strains. In this study, we tested whether ectopic expression of Bm-aaNAT and Bm-ebony interferes with the black melanin pigmentation of silkworms. Using the GAL4/UAS binary system, we found that ectopic expression of the Bm-aaNAT gene alters the coloration of neonatal larva from a dark ant-like color to light brown. In addition, overexpression of the Bm-aaNAT and Bm-ebony genes changed the pigmentation in the cuticle of second- to final-instar larva and the adult antennae from black/brown to a lighter color. We also demonstrate that expressing the Bm-aaNAT gene under the direct control of a constitutive baculovirus immediate early 1 ( IE1 ) gene promoter produced a color transformation in neonatal larvae. Furthermore, the Bm-aaNAT gene had ability to lighten dark melanin coloration in ladybird beetle H. axyridis and fruit fly D. melanogaster , which strongly indicates the utility of Bm-aaNAT gene as a dominant molecular marker in insects. Bm-aaNAT lightens body color of neonatal larvae in silkworm To express Bm-aaNAT and Bm-ebony in B. mori , we first used the binary GAL4/ upstream activating sequence (UAS) system. Effector vectors that carried the Bm-aaNAT gene or Bm-ebony gene linked to an UAS and an EGFP reporter gene under the control of the eye-specific 3xP3 promoter were constructed ( Fig. 1a ). The effector lines were generated by germline transformation. After sib mating and selection of G1 progeny based on the presence of EGFP fluorescence, G1 male moths were crossed with female moths of the actin A3 -GAL4 driver line 193-2, which drives ubiquitous expression of GAL4, and can be identified by the 3xP3-DsRed2 marker ( Fig. 1a ) [36] . The overexpression of Bm-aaNAT and Bm-ebony was first tested in the w1-pnd strain, which is generally used to produce transgenic silkworms because the white-egg phenotype is convenient for fluorescence screening of the embryonic eye. In contrast to the blackish coloration of control w1 neonatal larvae, the head and the body of the newly hatched larvae were light brown in color in all three actin A3 -GAL4; UAS- NAT lines ( Fig. 1b , Supplementary Fig. S1 online). This suggests that Bm-aaNAT interfered with the dopamine-melanin synthesis cascade in the cuticle of neonatal larvae, and produced NADA, leading to lighter melanin pigmentation. However, only a subtle change in coloration was observed in actin A3 -GAL4; UAS- ebony neonatal larvae ( Fig. 1c , Supplementary Fig. S1 ), although we checked several lines. 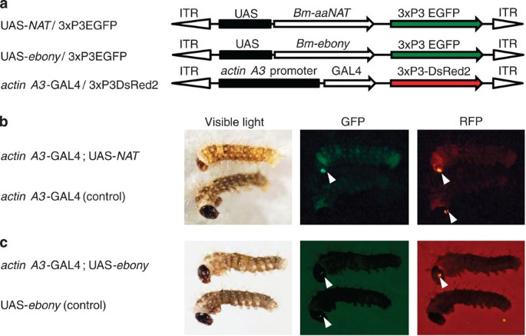Figure 1:Bm-aaNAToverexpression alters cuticle coloration in neonatal silkworm larvae. (a) Structures of UAS-NAT/3xP3EGFP, UAS-ebony/3xP3EGFP andactin A3-GAL4/3xP3DsRed2 (not to scale). 3xP3, eye-specific promoter; ITR, inverted terminal repeat of thepiggyBactransposon. Effect of ectopic expression ofBm-aaNAT(b) andBm-ebony(c) using the GAL4/UAS binary system (w1-pnd background). Left, bright field; middle, GFP; and right, red fluorescent protein (RFP). White arrowheads indicate fluorescence in the ommatidia. Figure 1: Bm-aaNAT overexpression alters cuticle coloration in neonatal silkworm larvae. ( a ) Structures of UAS- NAT /3xP3EGFP, UAS- ebony /3xP3EGFP and actin A3 -GAL4/3xP3DsRed2 (not to scale). 3xP3, eye-specific promoter; ITR, inverted terminal repeat of the piggyBac transposon. Effect of ectopic expression of Bm-aaNAT ( b ) and Bm-ebony ( c ) using the GAL4/UAS binary system (w1-pnd background). Left, bright field; middle, GFP; and right, red fluorescent protein (RFP). White arrowheads indicate fluorescence in the ommatidia. Full size image Bm-aaNAT and Bm-ebony suppress larval black pigmentation In wild-type silkworm strains, after the second instar, the epidermis is mainly white and opaque due to the accumulation of uric acid granules, and has several black markings consisting of melanin and ommochrome pigmentation. To observe the effects of ubiquitous overexpression of Bm-aaNAT and Bm-ebony in older instar larvae, we chose to use the black striped strain striped ( p S ; Fig. 2 ). This strain has a wide black stripe in each segment induced by the dominant striped gene p S , in addition to the melanin pigmentation in eyespot markings of the second thoracic segment, crescent markings in the second abdominal segment, and star spot markings in the fifth abdominal segment, which are present in wild-type strains. We crossed the striped gene p S homozygotes with actin A3 -GAL4; UAS- NAT and actin A3 -GAL4; UAS- ebony lines ( Supplementary Fig. S2 ). As expected, the ectopic expression of aaNAT caused marked changes in pigmentation although the coloration of each instar differed. In the both second- and the third-instar larvae of actin A3 -GAL4; UAS- NAT ( p S ) lines, the black body stripes, and the crescent and star spot markings on the second and fifth abdominal segments were a very light tan color ( Supplementary Fig. S3 ). In the fourth-instar larvae of these lines, the black body stripes were a light brownish grey color, and crescent markings and star spot markings were a lighter brown color. In addition, the brown-coloured area was larger compared with wild type, especially in the crescent markings ( Supplementary Fig. S4 ). In the fifth instar, the stripes were light grey instead of black ( Fig. 2 ). Notably, the pigmented areas of eyespot markings in the second thoracic segment, crescent markings, and star spot markings were markedly smaller and the shapes of the crescent and star spot markings were altered ( Fig. 2 ). These observations indicate that the ectopic expression of Bm-aaNAT not only affects the synthesis of melanin pigments in neonatal larvae, but throughout the larval stages. 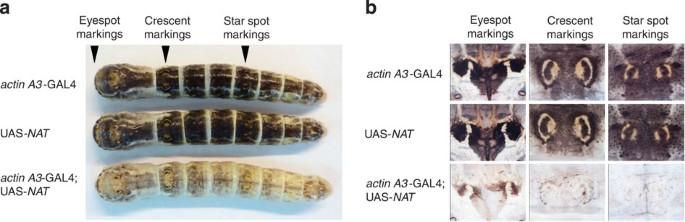Figure 2:Bm-aaNAToverexpression lightens pigmentation in the black striped silkworm strain. The fifth-instar larvae shown here have the dominantstriped(pS) genetic background. (a) Dorsal view of the larvae. The positions of the markings magnified inbare indicated by the arrowheads. (b) Magnified images of the larval markings. Figure 2: Bm-aaNAT overexpression lightens pigmentation in the black striped silkworm strain. The fifth-instar larvae shown here have the dominant striped ( p S ) genetic background. ( a ) Dorsal view of the larvae. The positions of the markings magnified in b are indicated by the arrowheads. ( b ) Magnified images of the larval markings. Full size image Although the actin A3 -GAL4; UAS- ebony showed no marked changes in neonatal larval coloration, a change in pigmentation was observed from the second instar in p S -crossed individuals. Like actin A3 -GAL4; UAS- NAT ( p S ) lines, larval pigmentation differed between stages, but was also different from aaNAT -overexpressing lines. The color of the markings in the second-instar larvae of actin A3 -GAL4; UAS- ebony ( p S ) lines changed from black to pale yellow. In the third-instar larvae, most of the black regions changed to a darker orange-yellow color, which was different from that in actin A3 -GAL4; UAS- NAT ( p S ) larvae of the same instar ( Fig. 3 ). Although black pigmentation was not observed in the third-instar larvae of actin A3 -GAL4; UAS- NAT ( p S ) lines, it remained in actin A3 -GAL4; UAS- ebony ( p S ) lines in several areas such as the margins of the crescent marking. In the fifth-instar larvae, ectopic ebony overexpression did not induce yellowish coloration, and the change of pigmentation was modest compared with that in younger larvae. However, they could be distinguished from non-overexpressing lines by the loss of pigmentation in the lateral area especially in areas surrounding the spiracles, and in the dorsal region of the second and third thoracic segments ( Supplementary Fig. S5 ). 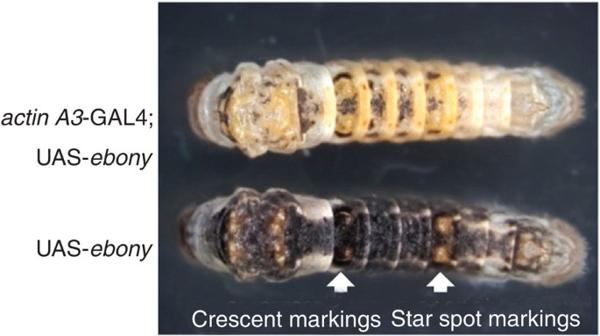Figure 3:Bm-ebonyoverexpression alters silkworm larval pigmentation in older instars. The black striped silkworm (pS) strain, which the effect on melanin pigmentation is easy to observe is used. The dorsal view of third-instar larvae is shown. Ubiquitous overexpression ofBm-ebonychanged most areas of black pigmentation. Figure 3: Bm-ebony overexpression alters silkworm larval pigmentation in older instars. The black striped silkworm ( p S ) strain, which the effect on melanin pigmentation is easy to observe is used. The dorsal view of third-instar larvae is shown. Ubiquitous overexpression of Bm-ebony changed most areas of black pigmentation. Full size image As the silkworm tracheae are also pigmented with black melanin, we inspected the tracheae of 3-day-old fifth-instar larvae of actin A3 -GAL4; UAS- NAT and actin A3 -GAL4; UAS- ebony lines, and found them to be pale brown in color, indicating that dopamine was converted into NADA or NBAD instead of dopamine-melanin ( Supplementary Fig. S6 online). Taken together, our data show that ectopic expression of Bm-aaNAT affected melanization of the epidermal cuticle in larvae of all stages and the tracheae, and that ectopic expression of Bm-ebony affected the melanization of the second- to fifth-instar larvae and the tracheae. Bm-aaNAT and Bm - ebony lighten adult antenna coloration No clear differences were observed between control insects and actin A3 -GAL4; UAS- NAT - and actin A3 -GAL4; UAS- ebony -carrying insects in the wing scales and body hair of adult silk moths, which are normally white. However, a distinct change in the color of the antennae was observed ( Fig. 4 ). In contrast to the normal brown pigmentation, the antennae of Bm-aaNAT - and Bm-ebony -overexpressing insects were light brown in color. This suggests that the pigment of the antennae in adult silk moths is derived from dopamine-melanin, which was converted into NADA and NBAD by ectopically expressed Bm-aaNAT and Bm-ebony , respectively. 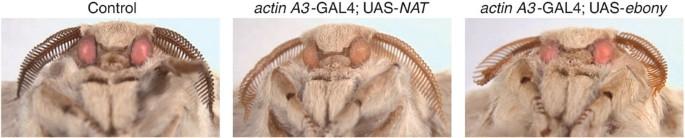Figure 4: Ectopic expression ofBm-aaNATandBm-ebonylightens adult antenna coloration. Moths carrying onlyactin A3-GAL4/3xP3DsRed2 were used as controls. Figure 4: Ectopic expression of Bm-aaNAT and Bm-ebony lightens adult antenna coloration. Moths carrying only actin A3 -GAL4/3xP3DsRed2 were used as controls. Full size image Development of a dominant marker with the Bm-aaNAT gene As the phenotype produced by ectopic Bm-aaNAT expression seemed to be ideal for a transformation marker, we next tested whether Bm-aaNAT directly linked to a promoter alters the black melanin coloration. We tested the B. mori actin A3 promoter and baculovirus IE1 gene promoter to drive expression of the transgene ( Fig. 5a ). Although no large difference in coloration was observed using the actin A3 promoter, the body color of neonatal larvae carrying the IE1 - NAT transgene was light brown ( Fig. 5b , left panel, white arrowheads, Supplementary Fig. S7 ) in all eight G1 strains expressing EGFP fluorescence in the eye, and the difference in color was easily distinguishable without the aid of a microscope. The transformation efficiency for IE1 - NAT transgene was 19% (8/43), which compared favourably with that achieved with the actin A3 -EGFP transgene (14%) and 3xP3EGFP transgene (12%) using the same system [37] . In addition, no significant difference was detected in the survival rate, and developmental time was only delayed for average of 1 day in IE1 - NAT G1 silkworms (average 81.3%, s.d.=15.1%, n =4) compared with their non-transgenic siblings (average 87.4%, s.d.=3.9%, n =4; P =0.47, Student’s t -test), and the subesequent generation also grew normally, and had no notable difference with non-transgenic siblings in fecundity ( Supplementary Fig. S8 , Supplementary Table S1 ). Furthermore, the light brown coloration was observed for larvae with 50% segregation obtained from an F1 backcross, which suggests that insertion of a single copy is enough to alter pigmentation. Moreover, when we used C146 (a commercial silkworm strain homozygous for the wild-type w1 ( kynurenine 3-mono oxygenase ) gene, which has brown ommochrome pigments in the epidermis in addition to melanin pigments; and 1.9-fold cocoon yield of w1-pnd strain, Supplementary Fig. S8 ), as the host for germline transformation, G1 transformants could easily be distinguished without microscopy by their orange-brown color ( Fig. 5b , right panel, white arrowheads), with only small decrease in cocoon weight ( Supplementary Fig. S8 ), verifying that the IE1 - NAT transgene can function as a dominant visible transgenic marker in practical wild-type silkworm strains. 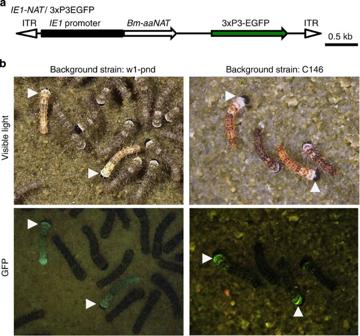Figure 5: Development of a dominant markerIE1-NATthat alters neonatal larval coloration. (a) Structure of theIE1-NAT/3xP3EGFP transgene.Bm-aaNATexpression was under the direct control of the constitutive baculovirusIE1promoter. (b) Neonate larvae carryingIE1-NATtransgene can be easily distinguished by its light coloration (white arrowheads), whether w1-pnd (kynurenine 3-mono oxygenase(KMO)-deficient strain, left panels) or commercial strain C146 (with intactKMOgene, right panels) is used as the host strain for transgenesis. Top panels, bright field; bottom panels, GFP filter. Figure 5: Development of a dominant marker IE1 - NAT that alters neonatal larval coloration. ( a ) Structure of the IE1 - NAT /3xP3EGFP transgene. Bm-aaNAT expression was under the direct control of the constitutive baculovirus IE1 promoter. ( b ) Neonate larvae carrying IE1 - NAT transgene can be easily distinguished by its light coloration (white arrowheads), whether w1-pnd ( kynurenine 3-mono oxygenase ( KMO )-deficient strain, left panels) or commercial strain C146 (with intact KMO gene, right panels) is used as the host strain for transgenesis. Top panels, bright field; bottom panels, GFP filter. Full size image Bm-aaNAT suppresses pigmentation also in other insect taxa Finally, to check the potential usefulness of Bm-aaNAT in diverse insect taxa, we tested heterologous expression of Bm-aaNAT in fruit fly D. melanogaster and ladybird beetle H. axyridis . First, we generated UAS- NAT effector fly lines with the same construct that used for silkworm, and crossed with heat shock protein 70 (hsp) -GAL4, and pannier -GAL4 (ref. 38 ) (which expresses GAL4 in a broad stripe along the dorsal midline of developing flies) lines. As a result, hsp -GAL4; UAS- NAT individuals had overall clearly lighter pigmentation and white bristles in the thoracic segment ( Fig. 6a ), and black pigmentation of pannier -GAL4; UAS- NAT individuals was diminished in the pannier expression domain ( Fig. 6b , bracket), in a similar manner to the pannier -GAL4; UAS- ebony phenotype reported by [12] (ref. 12 ). The light coloration phenotype was observed for both of the two UAS- NAT effector fly lines we obtained. These results indicate that the ectopic expression of Bm-aaNAT suppress black coloration also in Drosophila . For the ladybird beetle H. axyridis , we used the IE1 promoter and the Drosophila hsp promoter ( Supplementary Fig. S9A ) to drive Bm-aaNAT expression ( Fig. 6c ). Although the IE1-NAT transgene did not show any coloration effects, one of the three transgenic strains with hsp-NAT transgene produced markedly light-coloured larvae ( Fig. 6c , Supplementary Fig. S9B ), possibly due to the influence of a nearby enhancer. The light coloration phenotype of this strain was enhanced by heat shock treatment ( Fig. 6c ), and Bm-aaNAT expression was confirmed by reverse transcription–polymerase chain reaction ( Supplementary Fig. S9C ), supporting that the light coloration is caused by the effect of Bm-aaNAT . Overall, these results indicate that Bm-aaNAT has the ability to lighten melanin coloration also in several insect taxa other than Lepidoptera. 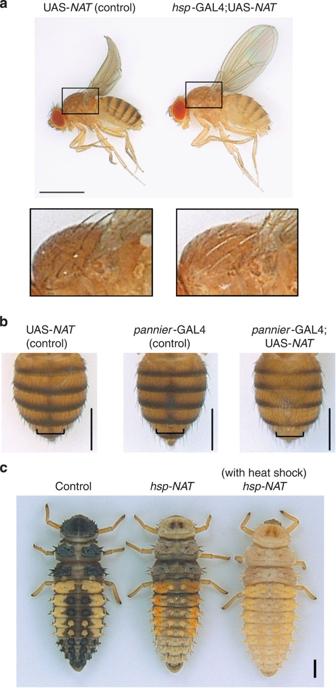Figure 6:Bm-aaNATlightens coloration in other insect orders. (a,b) Effect of ectopicBm-aaNATexpression inD. melanogaster. The flies are at least 4 days (100 h) old. Scale bar, 1 mm (a), 0.5 mm (b). (a) Shows the effect ofBm-aaNATdriven byhsp-GAL4. The fly shows overall lighter pigmentation, and as shown in the bottom panels (the magnified view of the square in the top panel) bristle coloration are also suppressed byBm-aaNAToverexpression. (b) Shows the effect ofBm-aaNATdriven bypannier-GAL4, which drives expression in a broad stripe along the dorsal midline (brackets). Abdomen of adult flies is shown. (c) Effect ofhsp-NATtransgene onH. axyridisfourth-instar larvae. Left, insect with no transgene; middle, insect withhsp-NATtransgene; right, insect withhsp-NATtransgene with heat shock treatment. Scale bar, 1 mm. Figure 6: Bm-aaNAT lightens coloration in other insect orders. ( a , b ) Effect of ectopic Bm-aaNAT expression in D. melanogaster . The flies are at least 4 days (100 h) old. Scale bar, 1 mm ( a ), 0.5 mm ( b ). ( a ) Shows the effect of Bm-aaNAT driven by hsp -GAL4. The fly shows overall lighter pigmentation, and as shown in the bottom panels (the magnified view of the square in the top panel) bristle coloration are also suppressed by Bm-aaNAT overexpression. ( b ) Shows the effect of Bm-aaNAT driven by pannier -GAL4, which drives expression in a broad stripe along the dorsal midline (brackets). Abdomen of adult flies is shown. ( c ) Effect of hsp-NAT transgene on H. axyridis fourth-instar larvae. Left, insect with no transgene; middle, insect with hsp-NAT transgene; right, insect with hsp-NAT transgene with heat shock treatment. Scale bar, 1 mm. Full size image We have shown that ectopic expression of Bm-aaNAT or Bm-ebony is sufficient to alter the black melanin pigmentation, which demonstrates their potential usefulness as dominant transformation markers. Although ubiquitous expression of Bm-aaNAT or Bm-ebony may affect the dopamine amount in the nervous system, there were no serious effects on fitness ( Supplementary Fig. S8 ) and behaviour such as eating and mating in the present experiments. In addition to facilitating the screening procedure, it is also beneficial regarding the choice of host strains for germline transformation. For instance, in silkworms, w1 mutant strain with white egg and eyes have been the feasible host for germline transformation because the eye-specific fluorescent markers are difficult to detect in wild-type strains with dark eggs and eyes. This has been a drawback for the analysis of most silkworm strains other than w1, and it is preferable to use commercial strains for production of biomaterials such as spider silk [39] because of their high productivity of silk. The use of aaNAT marker would be of benefit on such cases, and moreover, the widespread distribution of melanin-related pigments, conservation of the melanin synthesis pathway and ability of aaNAT to suppress black coloration even in flies and ladybird beetles ( Fig. 6 , Supplementary Fig. S9 ) suggest its potential as a transformation marker in diverse insect taxa. In the ladybird beetle, suppression of black pigmentation occurred only in the larval stage of a single strain out of three transgenic strains and was not observed in the adult stage, suggesting that the Bm-aaNAT expression in this strain is under the influence of a nearby enhancer. However, as the IE1 promoter is derived from Autographa californica polyhedrosis virus, it is likely that IE1 - NAT transgene could be directly applied to lepidopteran insects, which many species are known to be agricultural pests, and practical use of Bm-aaNAT gene should be possible for other taxa in combination with suitable promoters. Furthermore, aaNAT marker can be used in parallel with fluorescent markers because it does not interfere with the fluorescent signals, which enables the addition of an extra transgene. The data presented in this study also have significant impact for the understanding of molecular basis of melanin/cuticle synthesis. Although NADA is the most common precursor for colourless cuticle in the melanin/cuticle synthesis pathway of insects [22] , [23] , the gene involved in its synthesis had long remained unclear, until the recent discovery that Bm-aaNAT gene was disrupted in the B. mori mutant melanism [34] , [35] . Our results provide a direct evidence that Bm-aaNAT has the ability to lighten coloration in adults as well as the whole epidermal cuticle in silkworm larvae. Although Bm-aaNAT mutation in the mutant melanism has little effect on larval coloration, overexpression of Bm-aaNAT in this study induced marked changes throughout the larval stages ( Figs 1 , 2 , 4 , 5 , 6 , Supplementary Figs S1, S3, S4 and S7 online). The aaNAT gene was conserved in other lepidopterans such as monarch butterfly Danaus plexippus (GenBank accession code EHJ67891.1 ), and also was detected in 23 species out of 25 arthropods (excepting tick Ixodes scapularis and jewel wasp Nasonia vitripennis ) when searched by OrthoDB ( http://cegg.unige.ch/orthodb4 ). Recently, upregulated aaNAT expression linked with yellow pigmentation was reported in Heliconius butterfly hindwing [40] , which suggests that aaNAT functions as a modifier in melanin pigmentation of other insects. As for ebony , it has been described as a suppressor of black coloration in Drosophila that delimits the black pigmentation on the wing and abdomen [18] , [41] , and reported to change black melanin pigmentation to a tan color by ectopic expression ( Fig. 7 ) [18] . Ebony is also reported to be associated with the yellow/red pigments in the larval eyespot markings and adult wing of the swallowtail and Heliconius butterflies [40] , [42] , [43] , [44] . Our results showing that ectopic ebony expression alters the color of melanin pigments in larvae and adults are consistent with these reports, and the conservation of the ebony gene in arthropods (24 out of 25 species in OrthoDB, not detected only in I. scapularis ) suggest that it may contribute to light-coloured pigmentation in other lepidopterans. 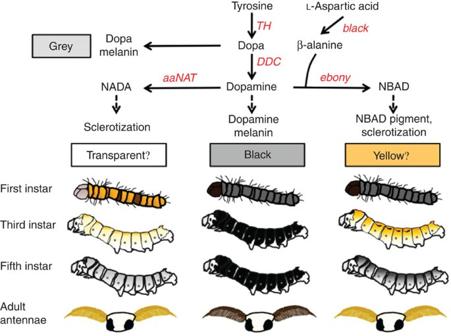Figure 7: Effects of overexpression ofBm-aaNATandBm-ebonyon silkworm pigmentation. ThestripedstrainpSis used in the model for larval coloration. The melanin synthesis pathway is adapted from Futahashiet al.16The melanic pigmentation of silkworm larvae and adult antennae is affected byBm-aaNATandBm-ebony, which use dopamine as substrate and produce transparent and yellowish cuticle, respectively. Notably,Bm-aaNATeffect on melanic pigmentation can be easily detected at the first instar, whereasBm-ebonydoes not have significant effect in this stage. TH, tyrosine hydoxylase; DDC, dopa decarboxylase. Figure 7: Effects of overexpression of Bm-aaNAT and Bm-ebony on silkworm pigmentation. The striped strain p S is used in the model for larval coloration. The melanin synthesis pathway is adapted from Futahashi et al. [16] The melanic pigmentation of silkworm larvae and adult antennae is affected by Bm-aaNAT and Bm-ebony , which use dopamine as substrate and produce transparent and yellowish cuticle, respectively. Notably, Bm-aaNAT effect on melanic pigmentation can be easily detected at the first instar, whereas Bm-ebony does not have significant effect in this stage. TH, tyrosine hydoxylase; DDC, dopa decarboxylase. Full size image Notably, ectopic expression of Bm-aaNAT and Bm-ebony had different effects in silkworm larvae. In general, Bm-ebony overexpression induced a more yellowish coloration than Bm-aaNAT in the black striped p S strain ( Fig. 7 ). This is consistent with the previous observations that cuticles sclerotized exclusively by NADA (product of aaNAT ) are colourless or very lightly straw-coloured, and grow darker brown the more NBAD (product of ebony ) dominates in the process ( Fig. 7 ) [23] . Furthermore, in contrast to the control silkworms whose markings were black throughout the larval stage, coloration differed between stages in Bm-aaNAT- and Bm-ebony- overexpressing silkworms ( Fig. 7 ). For example, p S larvae with ectopic Bm-aaNAT expression showed gold-brownish coloration in the third and fourth instars ( Supplementary Figs S3 and 4 online), and greyish coloration in the fifth instar ( Fig. 2 ). As both aaNAT and Ebony use dopamine as a substrate and do not affect the production of dopa-melanin, the differences in the coloration between larval stages may reflect the increase of grey dopa-melanin in the elder instars ( Fig. 7 ). In the control larvae, grey dopa-melanin may be concealed by black dopamine-melanin, leaving its presence undetectable. In the Bm-ebony -overexpressing larvae, more significant differences in coloration between larval stages and areas were observed. It is noteworthy that only a subtle color change was observed in neonatal larvae and some areas remained black in the third-instar larvae with Bm-ebony overexpression ( Figs 1 , 3 and 7 ). As β-alanine is required for the conversion of dopamine to NBAD by Ebony ( Fig. 7 ), a possible cause of these observations may be a difference in the uptake or accumulation of β-alanine. β-Alanine is produced by the action of the product of black gene ( Fig. 7 ) in D. melanogaster and T. castaneum , whose adult black mutants are dark and black, respectively [45] . In the silkworm, a previous microarray analysis shows that the black gene is not expressed in the first instar [46] , suggesting that ectopic Bm-ebony expression could not alter neonatal larval coloration because of lack of β -alanine. The ubiquitous effect of aaNAT may be because the widely abundant acetyl-coA is its cofactor for the conversion of dopamine to NADA. Until now, the ‘visible markers’ used for insect transgenesis were based on D. melanogaster mutants and mostly restricted to the same species, due to the lack of mutants to use as host strains in other insects. As pigmentation is realized by the action of many genes, a dominant molecular marker that produces pigments where they did not originally exist seemed to be challenging. Our experiments indicate that a ‘visible marker’ based on melanin pigments can be developed using the opposite approach, that is, by reducing pigmentation. As this strategy led to visible changes in larvae of all stages and even in adults, the aaNAT transgene should enable the screening of transgenic insects during most of their lifetime ( Fig. 7 ). The application of the aaNAT transformation marker should facilitate the use of transgenic techniques and promote molecular studies in insects. Insects The silkworm strains w1-pnd, actin A3 -GAL4/3xP3-DsRed2 ( w1 ) [47] and C146 are maintained at the Transgenic Silkworm Research Unit of NIAS, and the p S strain at the Genetic Resource Center of NIAS. Silkworms were reared at 25 °C with mulberry leaves or artificial diets (Nihon Nosan Kogyo, Yokohama, Japan) under a 16-h light: 8-h dark photoperiod. D. melanogaster was reared on a standard medium at 27 °C. The embryos used as recipients for DNA injection to generate transgenic lines were Oregon R. The GAL4 lines used in this study is as follows; hsp -GAL4 ( w[*]; P{w[+mC]=GAL4-Hsp70.PB}2/CyO ) and pannier -GAL4 (ref. 38 ) (y1 w1118; P{w+mW.hs=GawB}pnrMD237/TM3, P{w+mC=UAS-y.C}MC2,Ser1 ). H. axyridis was purchased from Agrisect Inc. (Japan) and maintained as described previously [5] , [48] . The insects were reared at 30 °C, and heat shock cycles were applied from second instar. One cycle consisted of heat shock at 40 °C 1 h followed by recovery at 30 °C for 5 h. Donor plasmid construction To construct the pBacUAS- NAT /3xP3EGFP plasmid, the Bm-aaNAT ORF was amplified from p50T pupal wing cDNA with the primers pBacMCS-UAS-BlnI-Kozak-BmNAT1-ORF-s (5′-GCCTAGTAGACCTAGAAAAATCAAAATGGCTGTTACAAGTACAAGAGGC-3′) and pBacMCS-UAS-BlnI-BmNAT1-ORF-a (5′-GTATGGCTGACCTAGTTACAGCTCCTTAATGTAGACCCTG-3′), using Phusion Hot Start II High-Fidelity DNA Polymerase (New England Biolabs). The resulting PCR product was gel purified using a QIAquick Gel Extraction Kit (Qiagen) and subsequently cloned into the Bln I site of pBacUASMCS-3xP3EGFP using In-Fusion HD Cloning Kit (Clontech). The sequence was confirmed by the Sanger method using an ABI3130xl Genetic Analyser (Applied Biosystems). The Bm-aaNAT ORF sequence is the same as that with GenBank accession no. DQ256382 . To construct the pBacUAS- ebony /3xP3EGFP plasmid, the Bm-ebony ORF was amplified from p50T pupal wing cDNA with the primers pBacMCS-UAS-BlnI-Kozak-Bm-ebony-ORF-s (5′-GCCTAGTAGACCTAGAAAAATCAAAATGGGCTCCTTGCCTCGCGT-3′) and pBacMCS-UAS-BlnI-Bm-ebony-ORF-a (5′-GTATGGCTGACCTAGTTAGTCCAAGGGTTTCCAGCAC-3′). Subsequent procedures are the same as described above. The sequence of the Bm-ebony ORF was the same as that for GenBank accession no. AB455231 . To construct the pBac IE1 - NAT /3xP3EGFP plasmid, the IE1 portion of pIEx-2 (Novagen) was amplified with the primers hr5-IE1-BglII-s (5′-CATTGCGTAGATCTCGCGTAAAAC-3′) and hr5-IE1-BlnI-a (5′-AAAAAAAACCTAGGTCACTTGGTTGTTCACGATC-3′) and ligated into the 6-kb portion of Bgl II- and Bln I-digested pBacUASMCS-3xP3EGFP. The resulting plasmid was named pBac- IE1 -3xP3EGFP. Next, the Bm-aaNAT ORF was amplified from pBacUAS- NAT /3xP3EGFP with the primers pBacIE1BlnIKozakBmNAT1ORF-s-2 (5′-AACCAAGTGACCTAGGAAAAATCAAAATGGCTGTTACAAGTACAAGAGGC-3′) and pBacMCS-UAS-BlnI-BmNAT1-ORF-a (5′-GTATGGCTGACCTAGTTACAGCTCCTTAATGTAGACCCTG-3′), and was subcloned into the Bln I site of pBac- IE1 -3xP3EGFP using an In-Fusion HD Cloning Kit. To construct the pBac- hsp - NAT /3xP3EGFP plasmid, the hsp promoter portion was amplified with the primers Dmhsp70p-BglII-s (5′-AAAAAAAAAGATCTAAGCTTCTAGAATCCCAAAACAAACTGG-3′) and Dmhsp70p-BlnI-a (5′-AAAAAAAACCTAGGGAATTCCCAATTCCCTATTCAGAG-3′), and p10 gene 3′ UTR (to enhance protein production [49] ) portion was amplified with primers p10-5′-BlnI-s (5′-AAAAAAAACCTAGGATGAATCGTTTTTAAAATAACAAATC-3′) and p10-3′-PstI-a (5′-AAAAAACTGCAGGTTAACTCGAATCGCTATCCAAG-3′), ligated into the 5.5-kb portion of Bgl II- and Pst I-digested pBacUASMCS-3xP3EGFP. The resulting plasmid was named pBac- hsp -3xP3EGFP. Next, the Bm-aaNAT ORF was amplified from pBacUAS- NAT /3xP3EGFP with the primers Syn21-NAT-s (5′-TTGGGAATTCCCTAGGAACTTAAAAAAAAAAATCAAAATGGCTGTTACAAGTACAAGAGGC-3′) and P10-NAT-a (5′-AACGATTCATCCTAGGTTACAGCTCCTTAATGTAGACCCTG-3′), and was subcloned into the Bln I site of pBac- hsp -3xP3EGFP using an In-Fusion HD Cloning Kit. Generation of transgenic insects Germline transformation of silkworms using the w1-pnd strain was conducted as described previously [50] . Transgenic silkworm generation using the C146 strain was conducted according to a previously described method [51] , with modifications. To prevent entering into diapause, eggs were treated with 20% HCl for 30 min at 25 °C 4 h after oviposition [51] . Donor and helper plasmid DNAs were injected into 476 eggs 30 min to 3 h after acid treatment. After injection, the embryos were incubated at 25 °C to allow them to hatch. The hatch rate for HCl-treated C146 eggs was 26% (125 out of 476) for injected eggs and ~90% without injection. G1 screening was conducted by visual inspection on day 1 of first instar and was confirmed by fluorescence microscopy. Germline transformation of D. melanogaster was conducted as described previously [52] , [53] , using Oregon R as the host strain. PiggyBac -mediated germline transformation of ladybird beetle H. axyridis was conducted as described by Kuwayama et al. [5] Transgene screening was conducted by fluorescence microscopy at first instar. Fitness assessment of IE1 - NAT silkworms For each experiment, non-transgenic siblings were used as control. Survival rate, percentage of eclosed adults compared with first-instar larvae; developmental time, amount of days it took from hatching to eclosion; fecundity, number of eggs laid per female within 24 h of separation from male; coccon weight, weight of coccon after removal of pupa. Expression analysis of Bm-aaNAT in H. axyridis Total RNA was isolated from H. axyridis larva just before third moult using ISOGEN (Nippon gene), and reverse transcribed with a random primer (N6) using the first-strand cDNA synthesis kit (GE Healthcare) as previously described [16] . PCR conditions for Bm-aaNAT and Ha-rp49 ( H. axyridis ribosomal protein 49 gene) were as follows: 35 cycles of 94 °C for 30 s, 55 °C for 30 s and 72 °C for 30 s. Primers used for PCR are as follows; Ha-rp49 no. 1 (5′-GCGATCGCTATGGAAAACTC-3′), Ha-rp49 no. 2 (5′-TACGATTTTGCATCAACAGT-3′), BmNAT1-F1 (5′-CTGCCGGAGACTTGTGACTC-3′) and BmNAT1-R2 (5′-CATCTTGTAATTGAGCCTCTC-3′). How to cite this article: Osanai-Futahashi, M. et al. A visible dominant marker for insect transgenesis. Nat. Commun. 3:1295 doi: 10.1038/ncomms2312 (2012).